Induced and natural variation of promoter length modulates the photoperiodic response ofFLOWERING LOCUS T FLOWERING LOCUS T ( FT ) regulates the floral transition in many plant species by integrating environmental seasonal signals and internal cues. Here we show that two interdependent regulatory regions are necessary and sufficient to convey photoperiod responsiveness to FT . While a minimal distance between the regulatory regions is required to fully suppress FT expression under short days, increased distance reduces promoter response to long days. Natural variation at FT creating promoter length differences is widespread, correlates with longitudinal and latitudinal clines and affects a promoter region physically interacting with both photoperiod control regions. Three major FT promoter variants correlate with differences in FT allele usage in F1 hybrids. We propose that FT variation in cis could be adaptive by conferring differences in FT transcriptional control ultimately translating to increased fitness. Many plant species communicate information on day length from leaves to the apical meristem via a conserved mobile protein, FLOWERING LOCUS T (FT) to control the transition from vegetative to reproductive growth [1] , [2] , [3] , [4] . In addition to photoperiod, other external and internal cues such as temperature, light quality, stress and age converge at the level of transcriptional regulation of FT and enhance, repress or bypass the response to photoperiod [2] , [5] . The correct timing of flowering strongly impacts fitness and FT contributes as a quantitative trait locus to differences in flowering time [6] , [7] , [8] . Unravelling the transcription regulatory code of FT is the basis for understanding the evolution of its transcriptional regulation. We previously showed that the 5.7-kb region upstream of the transcription start site (TSS) of FT was necessary to initiate FT expression in long day (LD) conditions and contained three sequence blocks, A , B and C conserved among Brassicaceae species [9] . Block A , corresponding to the proximal FT promoter contains functional cis -regulatory elements directly bound by CONSTANS (CO), a B-box and CCT-domain containing transcription factor responsible for photoperiod control of FT [9] , [10] , [11] . However, it is not clear why such a long promoter evolved to drive photoperiod-dependent expression in leaves considering that the median intergenic distance in Arabidopsis is 1.4 kb and that most functional promoters are considered to be no longer than 500 bp (refs 12 , 13 ). Here we show that Blocks C and A are necessary and sufficient to confer responsiveness to LD, while the intermittent sequences are required to suppress background expression in short days (SDs). Within the intermittent sequence, a novel control region, Block ID , was identified that physically interacts with both core photoperiod control regions. Natural variation caused by large insertion-deletions (indels) overlapping with Block ID is widespread and correlates with geographical clines. Three major FT promoter variants caused by indels show differences in allele usage in F1 hybrids. Furthermore, cis -regulatory variation at FT may contribute to overall fitness as indicated by the reanalysis of previously published common garden experiments for the relative contribution of FT variants to the trait. The minimal FT promoter contains two regulatory regions To test whether Block C functions as a distal enhancer, a 5.2-kb FT promoter ( 5.2kbFTp) without Block C was fused to either beta-glucuronidase ( GUS ) or FT complementary DNA (cDNA) and stably transferred into Col-0 and ft-10 mutant plants ( Fig. 1a ). In LDs, ft-10 plants carrying 5 .2kbFTp::FTcDNA construct (hereafter 5 .2kbFTp::FTcDNA / ft-10 ) did not flower earlier than the parental ft-10 line and the GUS signal was not detected in 5 .2kbFTp::GUS/ Col-0 lines in histochemical assays ( Fig. 1b,c ; Supplementary Fig. 1 ). FT messenger RNA was not detectable in the leaves of 5.2kbFTp::FTcDNA/ft-10 plants grown in LD at any time point during the day corroborating that presence of Block C is required for FT expression in leaves ( Fig. 1d ). Block C was fused to the minimal promoter of the Nopaline Synthase ( NOS ) gene ( minNOSp ) [14] to test its capability to act as a general enhancer ( Fig. 1a ). In transient bombardment assays with Arabidopsis leaves, adding Block C ahead of minNOSp ( BlockC+minNOSp ) increased the relative signal of a LUCIFERASE ( LUC ) reporter threefold ( Supplementary Fig. 2 ). However, BlockC+minNOSp::FTcDNA / ft-10 plants did not flower earlier than ft-10 mutants grown in LD ( Fig. 1b ). Likewise, BlockC+minNOSp failed to drive GUS reporter expression in stably transformed Col-0 plants ( Fig. 1c ). Taken together, the data indicate that although Block C acts as an enhancer in the transient assay, it is not functional in driving the expression of FT in a chromosomal context. 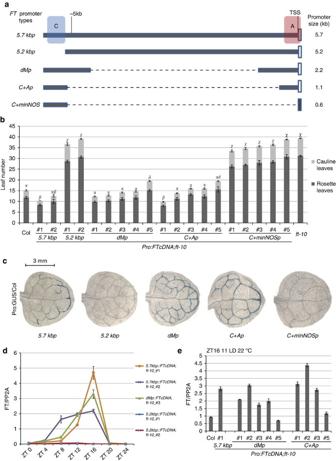Figure 1:Blocks CandAare necessary and sufficient forFTexpression in the leaf. (a) Schematic representation of differentFTpromoter constructs used in the analysis (TSS is +1). (b) Flowering time offt-10plants transformed withFTcDNA constructs driven by differentFTpromoters as depicted ina. Numbers of rosette and cauline leaves are shown as mean±s.e. Statistical significance was determined using one-way analysis of variance (ANOVA) and multiple comparison by the Holm–Sidak method (P<0.01). Different Greek symbols above the bars indicate significant differences. (c) Histochemical localization of GUS activity in the first true leaves of transgenic Col-0 expressingGUSgene under the control of differentFTpromoters as depicted ina. Leaves were collected at ZT16 after growth for 12 LDs on GM media. (d) Reverse transcriptase (RT)-qPCR analysis ofFTinft-10seedlings carrying the 5.7 kb, 5.2 kb ordMppromoter fused toFTcDNA. Seedlings were harvested from ZT0 to ZT24 on day 10 in LDs. Values represent mean±s.e. ofFTrelative toPP2Alevels for three technical replicates. A biological replicate showed similar results. (e) RT-qPCR ofFTinft-10seedlings carrying the5.7 kbp,C+ApordMppromoter fused toFTcDNA. Seedlings were harvested at ZT 16 on day 11 in LD conditions. Values indanderepresent mean±s.e. of relativeFTtoPP2Alevels for three technical replicates. A biological replicate showed similar results. Figure 1: Blocks C and A are necessary and sufficient for FT expression in the leaf. ( a ) Schematic representation of different FT promoter constructs used in the analysis (TSS is +1). ( b ) Flowering time of ft-10 plants transformed with FT cDNA constructs driven by different FT promoters as depicted in a . Numbers of rosette and cauline leaves are shown as mean±s.e. Statistical significance was determined using one-way analysis of variance (ANOVA) and multiple comparison by the Holm–Sidak method ( P <0.01). Different Greek symbols above the bars indicate significant differences. ( c ) Histochemical localization of GUS activity in the first true leaves of transgenic Col-0 expressing GUS gene under the control of different FT promoters as depicted in a . Leaves were collected at ZT16 after growth for 12 LDs on GM media. ( d ) Reverse transcriptase (RT)-qPCR analysis of FT in ft-10 seedlings carrying the 5.7 kb, 5.2 kb or dMp promoter fused to FT cDNA. Seedlings were harvested from ZT0 to ZT24 on day 10 in LDs. Values represent mean±s.e. of FT relative to PP2A levels for three technical replicates. A biological replicate showed similar results. ( e ) RT-qPCR of FT in ft-10 seedlings carrying the 5.7 kbp , C+Ap or dMp promoter fused to FT cDNA. Seedlings were harvested at ZT 16 on day 11 in LD conditions. Values in d and e represent mean±s.e. of relative FT to PP2A levels for three technical replicates. A biological replicate showed similar results. Full size image We used a promoter truncation approach to map the minimal promoter required for FT induction. A deletion of 3.5 kb ( dMp ) intermittent sequence within the 5.7-kb promoter or a direct fusion of Block A and Block C ( C+Ap ) driving FT expression resulted in transgenic ft-10 plants that flowered similar to Col-0 in LD ( Fig. 1a,b ), indicating that these shorter promoters responded normally to photoperiod. On the other hand, both truncated promoters extended the expression domain of the GUS reporter gene to the major veins compared with the 5.7kbFTp construct ( Fig. 1c ). This suggests that the region between Blocks C and A contains sequences involved in repressing FT , although the effect of derepression was not visible in the flowering time assay under LD conditions. Accordingly, if measured at the end of the day under LD conditions, FT levels were not significantly different in transgenic lines expressing FT under the control of 5.7kbFTp , dMp or C+Ap promoters ( Fig. 1d,e ). Variation in length alters FT promoter sensitivity Since the flowering time response in LD was not sensitive to small fluctuations in FT expression, we performed complementation experiments in growth conditions associated with reduced endogenous FT expression such as marginal long day (MD) and SD photoperiods as well as reduced ambient temperature. In any LD condition, independent lines containing dMp or C+Ap flowered as those carrying 5.7kbFTp::FTcDNA/ft-10 despite the differences in flowering time observed in plants grown at 30, 22 or 16 °C ( Fig. 2a ). However, under MD and SD, transgenic lines expressing FT under the control of shorter promoters flowered earlier compared with those carrying 5.7kbFTp ( Fig. 2a ). Indeed, GUS assays corroborated that dMp or C+Ap reporter lines show defects in FT repression since, in these plants, reporter activity was detected in the distal phloem of cotyledons and true leaves in SD, whereas 5.7kbFTp was fully repressed ( Fig. 2b ). 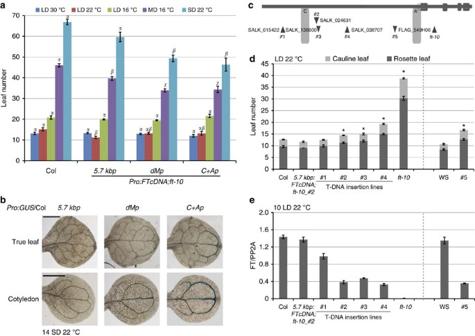Figure 2: Distance betweenBlock CandAmodifies the promoter response. (a) Flowering time offt-10plants expressingFTcDNA under the control of5.7 kb,dMandC+Apromoters in different growth conditions. Data were calculated based on two independent5.7 kb, threedMand threeC+Atransgenic lines. Col-0 was grown as control. Flowering time and statistical significance was determined as inFig. 1b. (b), Histochemical localization of GUS activity in the first true leaves and cotyledons of plants grown in 14 SDs at 22 °C. TheGUSreporter gene was driven by promoters5.7 kb, dMandC+Ain Col-0 background as indicated. Scale bars, 1 mm. (c,d) Flowering time was measured in LD-grown Arabidopsis plants carrying T-DNA insertions either upstream (#1) ofBlock Cor betweenBlock CandBlock A(#2–#5) at positions indicated by triangles. Line #5 is Ws and all other lines in the Col-0 accession. Statistical significance was determined pairwise for each genotype against the corresponding wild type using the Student’st-test (*P<0.01). Values represent mean±s.e. (n=12). (e) Reverse transcriptase-qPCR analysis ofFTtranscripts in the T-DNA lines shown inc. Seedlings were harvested at ZT16 on day 10 in LD conditions. Values represent mean±s.e. ofFTrelative toPP2Alevels of three technical replicates. A biological replicate showed similar results. Figure 2: Distance between Block C and A modifies the promoter response. ( a ) Flowering time of ft-10 plants expressing FT cDNA under the control of 5.7 kb , dM and C+A promoters in different growth conditions. Data were calculated based on two independent 5.7 kb , three dM and three C+A transgenic lines. Col-0 was grown as control. Flowering time and statistical significance was determined as in Fig. 1b . ( b ), Histochemical localization of GUS activity in the first true leaves and cotyledons of plants grown in 14 SDs at 22 °C. The GUS reporter gene was driven by promoters 5.7 kb, dM and C+A in Col-0 background as indicated. Scale bars, 1 mm. ( c , d ) Flowering time was measured in LD-grown Arabidopsis plants carrying T-DNA insertions either upstream (#1) of Block C or between Block C and Block A (#2–#5) at positions indicated by triangles. Line #5 is Ws and all other lines in the Col-0 accession. Statistical significance was determined pairwise for each genotype against the corresponding wild type using the Student’s t -test (* P <0.01). Values represent mean±s.e. ( n =12). ( e ) Reverse transcriptase-qPCR analysis of FT transcripts in the T-DNA lines shown in c . Seedlings were harvested at ZT16 on day 10 in LD conditions. Values represent mean±s.e. of FT relative to PP2A levels of three technical replicates. A biological replicate showed similar results. Full size image Since reducing the distance between Blocks C and A accelerated flowering under non-inductive conditions, we assessed whether enlarging the distance delayed flowering. We used several T-DNA lines carrying insertions immediately upstream of Block C (line #1) or between Block C and the TSS (lines #2–#5, Fig. 2c ). In LD and MD, line #1 flowered as early as the corresponding control Col-0, whereas lines #2–#4 clearly delayed flowering albeit not to the level of ft-10 mutants ( Fig. 2d ; Supplementary Fig. 3 ). This trend was also evident in line #5, which is in the Wassilewskija (Ws) background ( Fig. 2d ; Supplementary Fig. 3 ). The transcript levels of FT matched the flowering phenotype with a clear reduction at ZT16 in lines showing a delay in flowering ( Fig. 2e ). Taken together, an artificial increase in the distance between Block C and the TSS decreases the response of the FT promoter to inductive photoperiod, whereas a minimal distance between the regulatory elements is required to fully repress the promoter in non-inductive conditions. Three-dimensional structure of the FT locus The question arises on how the distal Block C communicates with Block A to participate in inducing FT transcription by photoperiod. We performed chromatin conformation capture (3C) assays to interrogate whether communication between regulatory regions of FT involves their physical interaction. In 3C, restriction fragments of cross-linked chromatin are ligated at a high dilution so that the ligation between physically attached fragments is strongly favoured over random ligation of non-attached fragments. Ligation frequencies between fragments are quantified by quantitative PCR and compared with the frequency of random ligation. When the restriction fragment including Block A and the TSS was used as a fixed point, a strong interaction with a region ~1.5 kb downstream of Block C , designated as Block ID , and a considerably weaker interaction with Block C were detected ( Fig. 3a,b ). The T-DNA line #2 inserted between Block C and ID reduced the interaction frequency for A–C but not for A–D ( Fig. 3b ). When 3C was carried out using Block ID as a fixed reference, interactions with Blocks A and C were confirmed ( Fig. 3c ). When Block C was used as a fixed region in 3C experiments, the interaction with Block ID was considerably stronger than that detected for the proximal promoter region ( Fig. 3d ), confirming the result obtained using Block A as a fixed point ( Fig. 3b ). Taken together, the intermittent promoter region ID interacts with Block A and Block C . In addition, the insertion of a T-DNA mostly abolished C–ID interactions and also reduced interaction of Block C with other parts of the promoter including Block A ( Fig. 3b ). 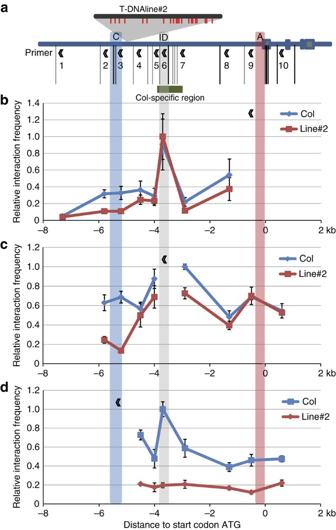Figure 3: Physical interaction betweenFTpromoter regions. (a) A high-resolution digestion map of theFTpromoter by the enzyme Sau3AI. Primers were designed on 10 restriction fragments as indicated.Blocks A,CandIDare indicated with red, blue and grey overlays, respectively. The green box indicates the location of an insertion present in the reference Col as compared to many re-sequenced accessions. The grey shadowing arrow indicates the insertion site of T-DNA mutant #2 with a digestion map indicated. At ZT16 after 10 days growth in LD, seedlings were collected for the 3C assay. Interaction frequency was corrected for primer and ligation efficiency usingBACF5I14 as control template after digestion and ligation. Values were scaled to set the highest interaction point per fixed primer to 1. Primer 9 (b), 6 (c) and 3 (d) were tested against all other primers to measure interactions. The position of the fixed primer is indicated by an arrow. Values are means of two biological replicates±s.e. Figure 3: Physical interaction between FT promoter regions. ( a ) A high-resolution digestion map of the FT promoter by the enzyme Sau3AI. Primers were designed on 10 restriction fragments as indicated. Blocks A , C and ID are indicated with red, blue and grey overlays, respectively. The green box indicates the location of an insertion present in the reference Col as compared to many re-sequenced accessions. The grey shadowing arrow indicates the insertion site of T-DNA mutant #2 with a digestion map indicated. At ZT16 after 10 days growth in LD, seedlings were collected for the 3C assay. Interaction frequency was corrected for primer and ligation efficiency using BAC F5I14 as control template after digestion and ligation. Values were scaled to set the highest interaction point per fixed primer to 1. Primer 9 ( b ), 6 ( c ) and 3 ( d ) were tested against all other primers to measure interactions. The position of the fixed primer is indicated by an arrow. Values are means of two biological replicates±s.e. Full size image Natural variation at FT Interestingly, Block ID colocalizes with a region showing structural variation among Arabidopsis accessions [6] , [15] . To assess whether structural polymorphisms in the FT promoter region could mediate variation in FT expression and flowering, we analysed natural molecular variation at FT by comparing a 6-kb region upstream of the start codon extracted from high-quality sequencing data from 81 Arabidopsis accessions [16] . This analysis confirmed the presence of two previously described promoter types [6] , [15] varying in size termed ‘long’, ‘medium’, and revealed a novel ‘short’ type ( Fig. 4a ; Supplementary Fig. 4 ). Phylogenetic analysis of the FT locus based on available single-nucleotide polymorphism (SNP) data revealed that the most frequent ‘medium’ form was ancestral and that the structural variation originated from at least two independent events: an insertion (~1.1 kb) and a deletion (~250 bp) around Block ID giving rise to the ‘long’ and ‘short’ promoters, respectively ( Fig. 4a,b ; Supplementary Figs 5 and 6 ). The 1.1-kb insertion region seems bipartite and is interrupted by a 140-bp sequence conserved in the ‘medium’ type that is in turn partially deleted in the ‘short’ type. Whereas the distal part of the insertion is of unknown origin, the proximal part consists largely of sequence nearly identical (97%) to a region on chromosome 5 ( Supplementary Fig. 7 ). Both inserted fragments contain insertion-site duplications indicating a transposase-mediatd origin, although the inserted sequences themselves are not related to known transposable elements ( Supplementary Fig. 7 ). 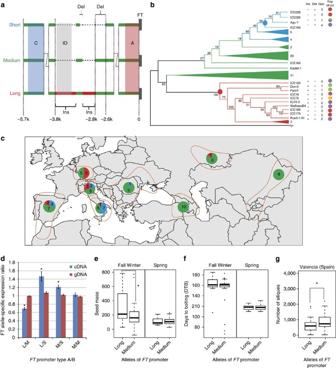Figure 4: Footprints of selection forFTpromoter variants. (a) Natural variation atFTpromoter. Insertions (Ins) and deletion (Del) are illustrated by the red boxes and horizontal dashed lines, respectively. Regions without prominent structural variation are shown as ‘zigzag’. (b) Maximum-likelihood phylogeny of the coding and promoter regions ofFTfrom 80 Arabidopsis accessions. Blue, green and red branches and collapsed clades denote short, medium and longFTpromoters, respectively.A. lyrata FTwas used as outgroup; bootstrap values shown at the nodes (%). Filled circles indicate sub-clades carrying footprints of selection. ‘Ins’, ‘Del’ and ‘Geo’ columns describe, respectively,FTpromoter variants and geographical origin. Pie charts illustrate population structure as previously determined16. (c) Geographical distribution ofFTpromoter variants. Distribution of ‘long’, ‘medium’ and ‘short’ variants across eight geographic areas16as pie charts coloured in red, green and blue, respectively, with numbers of accessions indicated. (d) Allele-specific expression ofFTin groups of F1 hybrids grown for 12 days in LD. L: ‘long’, M: ‘medium’ and S: ‘short’. Asterisk (*) indicates significant differences between cDNA and genomic DNA control (Student’st-test,P<0.01). Values represent mean±s.e. of six biological replicates. (e) Variation inFTpromoter length and fitness. The ‘long’ promoter contributes to more seed mass in fall–winter but not spring (data from Korveset al.17). Glm regression and non-parametric Wilcoxon rank sum test support a significant difference between ‘long’ and ‘medium’ promoters (*P<0.025). (f) Variation atFTpromoter does not alter flowering time. Flowering time determined as days to bolting (DTB)17shows no significant difference due toFTpromoter type. (g) Variation atFTpromoter explains fitness variation in Spain. Common garden experiments (from Fournier-Levelet al.18) at four different European sites were re-analysed for 82 accessions with confirmedFTpromoter type and available high density SNP data3. The ‘medium’ slightly outperforms the ‘long’FTpromoter in silique production. The ‘short’ variant is removed from (e–g) as only three accessions were present in the datasets. Boxes in (e–g) represent the interquartile range, the line indicates the median. Data points extending more than 1.5 times the interquartile range are treated as outliers. Figure 4: Footprints of selection for FT promoter variants. ( a ) Natural variation at FT promoter. Insertions (Ins) and deletion (Del) are illustrated by the red boxes and horizontal dashed lines, respectively. Regions without prominent structural variation are shown as ‘zigzag’. ( b ) Maximum-likelihood phylogeny of the coding and promoter regions of FT from 80 Arabidopsis accessions. Blue, green and red branches and collapsed clades denote short, medium and long FT promoters, respectively. A. lyrata FT was used as outgroup; bootstrap values shown at the nodes (%). Filled circles indicate sub-clades carrying footprints of selection. ‘Ins’, ‘Del’ and ‘Geo’ columns describe, respectively, FT promoter variants and geographical origin. Pie charts illustrate population structure as previously determined [16] . ( c ) Geographical distribution of FT promoter variants. Distribution of ‘long’, ‘medium’ and ‘short’ variants across eight geographic areas [16] as pie charts coloured in red, green and blue, respectively, with numbers of accessions indicated. ( d ) Allele-specific expression of FT in groups of F1 hybrids grown for 12 days in LD. L: ‘long’, M: ‘medium’ and S: ‘short’. Asterisk (*) indicates significant differences between cDNA and genomic DNA control (Student’s t -test, P <0.01). Values represent mean±s.e. of six biological replicates. ( e ) Variation in FT promoter length and fitness. The ‘long’ promoter contributes to more seed mass in fall–winter but not spring (data from Korves et al . [17] ). Glm regression and non-parametric Wilcoxon rank sum test support a significant difference between ‘long’ and ‘medium’ promoters (* P <0.025). ( f ) Variation at FT promoter does not alter flowering time. Flowering time determined as days to bolting (DTB) [17] shows no significant difference due to FT promoter type. ( g ) Variation at FT promoter explains fitness variation in Spain. Common garden experiments (from Fournier-Level et al . [18] ) at four different European sites were re-analysed for 82 accessions with confirmed FT promoter type and available high density SNP data [3] . The ‘medium’ slightly outperforms the ‘long’ FT promoter in silique production. The ‘short’ variant is removed from ( e – g ) as only three accessions were present in the datasets. Boxes in ( e – g ) represent the interquartile range, the line indicates the median. Data points extending more than 1.5 times the interquartile range are treated as outliers. Full size image Natural variation at Block ID is functional The observation that both the insertion(s) and deletion independently targeted the region that is in close contact to both key photoperiod regulatory blocks suggests functional significance for FT regulation. The distribution of promoter variation at the FT locus across accessions revealed that either all three or two alleles were present within several rather distantly related populations [16] ( Supplementary Table 1 ). This suggests that natural selection may have maintained FT alleles in response to adaptive constraints ( Fig. 4b ). We associated diversity of FT with geographic coordinates ( Fig. 4c ; Supplementary Fig. 8 ). While the differential distribution of FT alleles along longitude could not be separated from geographical clines owing to population structure, the ‘short’ and ‘long’ FT promoter variants associated with respectively lower and higher latitudes, independently of population structure ( Supplementary Fig. 8 ; Supplementary Table 1 ). The ‘long’ FT promoter tends to accumulate in more Northern latitudes as compared with the ‘medium’ promoter type ( Supplementary Fig. 8 ; Supplementary Table 1 ). To test whether variation in the promoter regions is functional, we assessed allele-specific expression in F1 hybrids of 14 crosses (2 ‘long’ × ‘medium’, 2 ‘long’ × ‘short’, 3 ‘medium’ × ‘short’ and 7 ‘medium’ × ‘medium’) grown in LD conditions ( Supplementary Table 2 ). The ‘short’ promoter was the least responsive compared with ‘long’ or ‘medium’ types, indicating that the deletion within Block ID modulated its function negatively ( Fig. 4d ). Comparison of ‘long’ and ‘medium’ promoters revealed the former to be less expressed ( Fig. 4d ). Evidence for an ecological significance of FT promoter variants came from the analysis of available fitness data from 82 accessions with known FT promoter types grown in field studies in Rhode Island either as annual spring or biannual autumn cohorts [17] . The ‘long’ promoter type was associated with a fitness advantage when plants were grown over winter, but was without effect when plants germinated in spring ( Fig. 4e ; Supplementary Table 3 ). Although these experiments did not interrogate fitness of Arabidopsis accessions in their natural habitat in Western Europe, the data indicate that the effect of structural variation at FT is linked to particular environmental conditions. It is tempting to speculate that both FT variants, which appear to be slightly less expressed than the ‘medium’ allele, prevent precocious flowering in particular conditions. However, flowering time measured in the same study [17] as days to bolting was not significantly altered depending on the FT promoter type ( Fig. 4f ; Supplementary Table 4 ). This is also confirmed by the analysis of data from a different ecological study that probed fitness traits across common gardens at four different European locations [18] . In this study, the possible fitness advantage of possessing a particular FT promoter variant was much harder to detect and was only borderline significant for plants grown in Southern Spain, whereas it was not significant in Germany or the United Kingdom ( Supplementary Fig. 9 ; Supplementary Table 5 ). Taken together, the data indicate that three structural FT promoter variants created by at least two independent indel events targeting an overlapping region are maintained within Arabidopsis populations and correlate with subtle differences in FT responsiveness to inductive signals. Furthermore, in particular habitats and climatic conditions the variants may contribute to overall fitness. We have shown that the minimal photoperiod-responsive unit of FT promoter is composed of elements from two regulatory regions separated by a non-responsive intermittent region of variant length in Arabidopsis accessions (4.7−3.8 kb). The distal regulatory region, Block C , acts as a general enhancer in transient assays and is able to increase the base-line expression of a reporter gene driven by the pNOS minimal promoter. In contrast, in stably transformed plants, Block C requires the FT proximal promoter ( Block A ) as an obligatory partner to induce transcription in response to LD ( Fig. 1 ; Supplementary Fig. 1 ). We propose that a different chromatin context in the two experimental systems explains the seemingly contradicting observations. In stably transformed cells, the distal Block C may not only recruit transcriptional activators but also chromatin-dependent repressors, which require the sequence context of Block A for neutralization. In a previous study, we showed that Block A is sufficient for induction by CO in transient assays, but not in stably transformed cells [9] . Several cis -elements within Block A and a CCAAT -box within Block C have previously been shown to participate in FT induction by LD [9] , [10] , [19] . It will be interesting to see in future studies whether a combination of such a limited number of cis -elements is sufficient to reconstruct the LD-induced FT regulon in an artificially designed promoter. Data generated using analytical promoter reporter constructs and T-DNA insertion lines indicate that the distance between the FT regulatory regions modulates the response to photoperiod ( Figs 1 and 2 ). Deletion of the intermittent regions causes an increased background expression in the non-inductive photoperiod that translates into accelerated flowering in these conditions. In contrast, earlier flowering and increased FT expression is not observed in LD for FT promoters with deletions in the intermittent sequence. The opposite, a reduction of FT expression and delayed flowering in LD is observed if the distance between the regulatory regions is increased by insertion of T-DNAs within the intermittent region ( Fig. 2 ). We show that the FT locus folds into a three-dimensional structure that favours the interaction of both regulatory blocks with a third region, Block ID , within the intermittent promoter sequence ( Fig. 3 ). We propose that interaction of both regulatory regions with Block ID promotes physical contact between Blocks A and C , which is required to promoter expression. If the intermittent sequence is fully deleted, presence of Block ID is not required to promote proximity, whereas an increased distance decreases interaction frequency and thereby promoter efficiency. Interestingly, Block ID overlaps with a region showing structural variation caused by large indels in Arabidopsis accessions. Three major variants are found in 80 European accessions for which high-quality sequencing data have been recently published [16] . The shortest and longest variants derived independently from the ancestral promoter, which remains the most frequent variant across all populations. The longest version, such as present in the Col-0 reference genome, appears to have been created by two independent insertions events causing a 0.8-kb increase in distance between Blocks C and A ( Fig. 4 ). Both inserted fragments contain insertion-site duplications indicating a transposase-mediated origin, although the inserted sequences themselves are not related to known transposable elements ( Supplementary Fig. 7 ). Currently, it is unknown whether such fragment shuffling is exceptional for the FT locus or commonly observed in the Arabidopsis genome, which could be indicative of a novel mechanism of creating genome diversity. Several lines of evidence indicate that naturally occurring promoter variants create functional diversity. First, subtle changes in allele-specific expression between the three common promoter variants indicate that these increase the response spectrum of FT alleles to LD signals ( Fig. 4 ). Second, the association of two FT alleles with differences in fitness in common garden experiments [17] , [18] argues for an adaptive advantage of one allele over the other in particular growth conditions ( Fig. 4 ). The long FT promoter allele associated with increased fitness in an overwintering cohort grown in Rhode Island correlated with decreased fitness in an independent experiment carried out in Spain [18] , although in the latter case the increase in total seed production was only borderline significant ( Supplementary Fig. 9 ). We found a latitudinal cline in FT promoter-variant distribution in the European accessions with the shortest form accumulating in Southern and the longest version in more Northern latitudes, but performance differences between long and medium FT promoter variants were not evident when plants were grown in more Northern locations in Germany and the United Kingdom ( Fig. 4 ; Supplementary Fig. 8 ). One possible explanation is that within a comparable latitude range, a parameter not captured in available field studies determines whether FT promoter variants convey a fitness advantage. In particular, better fitness integrated over a sufficient number of years reflecting adaptation to variant microclimatic conditions are almost impossible to capture experimentally. Possibly, long-term artificial selection experiments starting with a defined number of near-isogenic lines could give the answer whether small differences in FT responsiveness are sufficient to favour one allele over the other at specific locations. Intriguingly, flowering time, expressed as days to bolting, was not significantly influenced by the presence of different FT alleles, although this gene is thought to be the key regulator of flowering time. However, several recent reports have revealed that FT plays a more general role in shaping plant growth traits, such as speed of outgrowth of lateral shoots [20] , number of branches initiated after the transition [8] and stability of the inflorescence [21] , all of which are likely to influence fruit production after the floral transition. Thus, it is possible that the fitness advantage conferred by a subtle change in FT expression may be disconnected from FT’s role in the timing of the floral transition. Taken together, our data indicate that a requirement for tight control of background expression required a physical separation of Block C and Block A , which are the two core regulatory regions required and sufficient for photoperiod and tissue-specific control of FT expression. The intermittent promoter region, in particular, Block ID seems to play a role in mediating communication between Blocks A and C . Furthermore, the necessity to fine-tune the response to photoperiod in different growth habitats has led to the accumulation of three FT promoter structural variants among natural Arabidopsis populations. Most importantly, future field studies are required to clarify whether and how variation at the FT promoter contributes to microadaptation. Plant growth For gene expression analysis and GUS histochemical assays, seeds were sterilized in 75% ethanol and sowed on GM medium supplemented by 1% sucrose. After stratification (4 °C, 3 days), plants were grown in climate chambers at 22 °C in LDs (16 h light/8 h dark) or SDs (8 h light/16 h dark). Time of transfer to climate chambers represents day 0. ZEITGEBER TIME (ZT) indicates time after light on. Ten-day-old seedlings were collected for RNA isolation. For flowering time measurements, seeds were sowed on soil and transferred to LDs, SDs or MDs (12 h light/12 h dark) after stratification (4 °C, 3 days). Percival cabinets were set to temperatures ranging from 30 to 16 °C as indicated. Rosette and cauline leaves in the main shoot were counted to determine flowering time. Statistical analysis was performed using one-way analysis of variance followed by multiple comparison by the Holm–Sidak method ( P <0.01) for multiple comparisons or by the Student’s t -test for paired comparisons as indicated. Plasmids construction and generation of transgenic plants Transgenic 5.7kbp:FTcDNA/ft-10 and 5.7kbp:GUS/ft-10 plants were previously described [9] . Block C and 5.2kbp were amplified using primer pairs BlockC-GW-FW/BlockC-GW-RE and 5.2kbFTp-GW-FW/1kbFTp-GW-RE, respectively. C+Ap was amplified by overlap PCR with primers BlockC-GW-FW/BlockC-overlapA-RE and BlockA-overlapC-FW/1kbFTp-GW-RE. Primer sequences are indicated in Supplementary Table 5 . Block C , 5.2kbp and C+Ap were introduced into vector pDONR207 (Invitrogen) by BP reaction. dMp was obtained by deleting a 3.5-kb region from 5.7kbFTp-pDONR207 by partial restriction enzyme digest with Eco RV and Ale I. 5.2kbp and C+Ap and dMp were introduced into GW-FTcDNA-pGREEN and GW-GUS-pGREEN destination vectors by LR recombination as described [9] . Block C was fused to minNOSp by LR reaction after creating a destination vector inserting minNOSp into GW-FTcDNA (or GUS or GreenLUC )- pGREEN vectors at the Hin d III cloning site. Transgenic plants were generated by Agrobacterium tumefaciens -mediated transfer of T-DNA using the floral dip method [9] . T-DNA insertion mutants ft-10 is a GABI-KAT line with a T-DNA inserted in the first intron of FT . T-DNA SALK lines #1–4 were collected from NASC in Columbia background and the insertion positions of T-DNA were between conserved Blocks C and A (SALK_015422, SALK_024631, SALK_136600, SALK_038707, respectively). Line #5 in Wassilevskija background also harbours a T-DNA inserting into the region between Blocks C and A (FLAG_549H06). Transient bombardment Gold particles (3 μg) were prepared for each bombardment. Gold particles were washed in 70% ethanol and sterile water and resuspended in 50% sterile glycerol. Five microgram of each Prom::GreenLUC-pGREEN and 35S prom ::RedLUC-pJAN DNA were mixed with 50 μl gold beads, 50 μl 2.5 M CaCl 2 and 20 μl 0.1 M spermidine. After two washes with 100% ethanol, the DNA–gold mix was resuspended in 50 μl 100% ethanol and used for two parallel bombardments of 5–10 mm Arabidopsis leaves using the Biolistic Particle Delivery System (Bio-Rad, PDS-1000/HE). After 12–24 h incubation in LD, luciferin (1 mM) was sprayed on the leaves and the emitted light was immediately measured with a charge-coupled device-camera adapted with optical filters to detect RedLUC or GreenLUC signals independently. The ratio of GreenLUC/RedLUC signals was calculated with the excel macro Chroma-LUC Calculator version 1.0 (Promega). Quantitative reverse transcriptase-PCR Total RNA was isolated according to the RNeasy Mini kit (Qiagen, Cat. no. 74104). Total RNA (5 μg) was treated with DNA-free Dnase I (Ambion, Cat. no. AM1906) and cDNA was generated at 42 °C for 2 h using Superscript II reverse transcriptase and T18 oligonucleotide for priming (Life Technologies, Cat. no. 18080-044). Quantitative PCR was performed in a real-time PCR cycler (Roche LC480). Ten-microlitre PCR reactions included ~50 ng cDNA, 10 pmol forward and reverse primer and 5 μl 2 × SYBR Green quantitative PCR buffer (Bio-Rad, Cat. no.18080-044). The expression data were calculated based on standard curves or delta Ct values. GUS histochemical staining Young seedlings were collected at ZT 16 after growth for 12 LDs or ZT 4 after 14 SDs. Samples were incubated in 90% acetone on ice for 30 min, rinsed with 50 mM sodium phosphate buffer and incubated for 24–36 h at 37 °C in GUS-staining solution (0.5 mg ml −1 X-Gluc, 50 mM sodium phosphate buffer, 0.5 mM potassium ferrocyanide, 0.5 mM potassium ferricyanide and 0.1% Triton X-100). After incubation, samples were washed with 50 mM sodium phosphate buffer for 30 min and 70% ethanol several times until leaves turned white. The GUS staining was visualized and photographed under the stereomicroscope (Leica). Chromosome Conformation Capture (3C) Ten-day-seedlings (3 g) grown on soil were collected and infiltrated with 1 × phosphate-buffered saline with 2% formaldehyde under vacuum for 20 min. Glycine (0.1 M) was added to quench formaldehyde. Seedlings were ground in liquid N 2 and resupended in 50 ml nuclei isolation buffer (20 mM Hepes pH 8.0, 250 mM sucrose, 1 mM MgCl 2 , 5 mM KCl, 40% glycerol (v/v), 0.25% Triton X-100 (v/v), 0.1% 2-mercapto-ethanol (v/v), 1 × Proteinase Inhibitor Cocktail (Roche)), filtered through two layers of nylon mesh (70 μm and 40 μm) and pelleted at 3,000 g for 20 min at 4 °C. Nuclear pellets were washed once in 1 ml 1 × restriction enzyme buffer and then resuspended in 500 μl 1.2 × restriction enzyme buffer (New England Biolabs) with 0.15% SDS. After incubation at 900 r.p.m. for 40 min at 37 °C and 20 min at 65 °C, Triton X-100 was added to 2% to sequester SDS. Incubation was continued at 900 r.p.m. for 60 min at 37 °C. Next, chromatin DNA was digested for 20 h at 37 °C with Sau3AI (500 U) while agitating at 900 r.p.m. To inactivate Sau3AI, 1% SDS was added for 10 min at 65 °C. For ligation, 700 μl digested nuclei were incubated in a final volume of 5 ml, corresponding to a DNA concentration of 0.7 ng μl −1 , in 1 × T4 DNA ligation buffer (New England Biolabs) in the presence of 1% Triton X-100 for 5 h at 16 °C using 1000 U T4 DNA ligase (New England Biolabs), followed by 45 min incubation at room temperature. De-crosslinking was carried out by overnight incubation at 65 °C in the presence of 40 μg ml −1 proteinase K. Finally, 3C ligation products were purified by phenol:chloroform:isoamylalcohol (25:24:1) extraction. Precipitated DNA was dissolved in 200 μl H 2 O. In parallel, BAC clone F5I14 was digested and ligated. 3C DNA ligation products were quantified by real-time PCR and normalized to BAC control using the—delta delta Ct method (see Supplementary Table 6 for PCR primers). Allele-specific expression in F1 hybrids PCR primers flanking the SNP (G/C) in exon 4 distinguishing FT alleles in F1 hybrids were manually designed (see Supplementary Table 6 ). Reverse primers were biotinylated to purify PCR products using streptavidin beads (GE Healthcare). For each F1 plant, genomic DNA was isolated from two leaves of seedlings grown 12 days in LD on soil using Plant DNAeasy kit (Qiagen) according to the manufacturers’ instructions. The remaining shoot was used for RNA isolation using the RNAeasy kit (Qiagen). Following reverse transcription using Superscript II reverse transcriptase (Invitrogen) according to the manufacturers’ instructions, cDNA and genomic DNA were PCR amplified using the following conditions: 94 °C for 2 min; 50cycles of 94 °C for 30 s; 58 °C for 30 s; 72 °C for 45 s; 72 °C for 10 min. The PCR products were bound to streptavidin beads and transferred into 40 μl of annealing buffer (Qiagen, no. 979009) containing 10 pmol sequencing primer. The mixture was heated at 80 °C for 2 min and then cooled to room temperature. Amplicons were sequenced using a Qiagen Pyrosequencer PSQ 96MA following the manufacturer’s protocol for vacuum sample preparation and pyrosequencing reactions. SNP ratios were determined by quantifying the ratio of polymorphic peaks to monomorphic controls. Six individual plants were measured for each F1 hybrid. Phylogenetic analysis and footprints of selection The region of Arabidopsis chromosome 1 (24325426-24333934) comprising the full-length FT gene (AT1G65480; NC_003070.9) and the 6-kb upstream promoter region was extracted from the ‘genome matrix’ representing aligned genomes of 81 Arabidopsis accessions [16] ( http://1001genomes.org/data/MPI/MPICao2010/releases/current/genome_matrix/TAIR10_genome_matrix_2012_03_13.txt.gz ). Corresponding sequence of the A. lyrata FT locus was extracted from NCBI GenBank (NW_003302554: 9486908-9495749) and used as an outgroup in the phylogenetic analyses. All non-ATGC characters were treated as gaps and excluded from the phylogenetic analyses. The alignment was converted from fasta to Phylip4 format using ReadSeq 2.1.30 tool implemented at EBI ( http://www.ebi.ac.uk/cgi-bin/readseq.cgi ). A best-scoring maximum-likelihood tree was calculated using the fast bootstrapping algorithm (1,000 replicates) of the RAxML 7.3.5 with the GTRGAMMA model and the random seed numbers ‘−p’ and ‘−x’ set to 32,149 and 45,6789, respectively [22] . The tree was edited in Dendroscope 3 (ref. 23) [23] and Adobe Illustrator 11.0.0 software. The geographic regions and population structure of the genotypes were as described by Cao et al . [16] The Median Joining haplotype network was constructed using SplitsTree4 with default parameters [24] . The clinal association of the ‘long’, ‘medium’ and ‘short’ FT clades with the geographic coordinates was tested using pairwise Student’s t -tests. Statistical analysis of FT promoter variation with fitness We compiled seed mass and bolting time data from Korves et al . [17] and fruit production and survival data from Fournier-Level et al . [18] for accessions with PCR-confirmed FT promoter polymorphisms. In the Korves data set, 26 accessions were shown to carry the long, 53 accessions the medium genotype and three the short promoter type by PCR. In the Fournier-Level data set, 24, 52 and 3 accessions carried long, medium and short promoters, respectively. We used principal component coordinates to control the population structure [25] by analysing the 250 K SNP data set provided by Atwell et al . [26] The first 10 principal coordinates (PC1 to PC10), which can explain about 50% of the total genetic variation, were incorporated into a statistical model to analyse the effect of FT genotypes on each of the phenotypes. To calculate the significance of associations of FT promoter types with geographical clines, we used population structure parameters provided by Cao et al . [16] All statistical analyses were performed using the glm function in R and included the FT promoter type (long, medium and short), FRI functionality (functional (F) and non-functional (N)) experimental season in the Korves data set or experimental location in Fournier-Level data set, and 10 PCs. We performed model reduction by removing non-significant interaction following the procedure and suggestions by Crawley [27] . The likelihood ratios for models with and without interaction item were compared and tested by the χ 2 -method using the R-function analysis of variance. A non-parametric Wilcoxon rank sum test was applied to test the significance of differences between long and medium FT promoter types. This test showed the same significant trend as the glm regression assay. Only three accessions of the short genotype had been scored for fitness, reducing the statistical power to test predictions made for this variant. How to cite this article: Liu, L. et al . Induced and natural variation of promoter length modulates the photoperiodic response of FLOWERING LOCUS T . Nat. Commun. 5:4558 doi: 10.1038/ncomms5558 (2014).